β-Arrestin1 enhances hepatocellular carcinogenesis through inflammation-mediated Akt signalling G-protein-coupled receptors (GPCR) constitute the largest known superfamily for signal transduction and transmission, and they control a variety of physiological and pathological processes. GPCR adaptor β-arrestins (ARRBs) play a role in cancerous proliferation. However, the effect of ARRBs in inflammation-mediated hepatocellular carcinogenesis is unknown. Here we show that ARRB1, but not ARRB2, is upregulated in inflammation-associated hepatocellular carcinoma (HCC) and paracancerous tissues in humans. A genotoxic carcinogen, diethylnitrosamine (DEN), significantly induces hepatic inflammation, TNF-α production and ARRB1 expression. Although ARRB1 deficiency does not affect hepatic inflammation and TNF-α production, it markedly represses hepatocellular carcinogenesis by suppressing malignant proliferation in DEN-treated mice. Furthermore, TNF-α directly induces hepatic ARRB1 expression and enhances ARRB1 interaction with Akt by binding to boost Akt phosphorylation, resulting in malignant proliferation of liver cells. Our data suggest that ARRB1 enhances hepatocellular carcinogenesis by inflammation-mediated Akt signalling and that ARRB1 may be a potential therapeutic target for HCC. Hepatocellular carcinoma (HCC), the main form of liver cancer, is the sixth most common cancer and the third most frequent cause of cancer death worldwide [1] . The exact mechanism of HCC initiation and development is still unclear, though inflammation has been shown to play a key role in this progression [2] . Inflammation-induced liver injury is a critical factor in the development of HCC. Two classes of inflammatory response induce liver injury; one is virus hepatitis or microbial attack resulting in persistent inflammation and the other is alcohol abuse, nonalcoholic steatohepatitis and drug-induced liver injury, which are associated with sterile inflammation. Hepatocellular carcinogenesis has a strong connection with chronic hepatitis infection, induced by both hepatitis B and C virus, alcohol abuse or non-alcoholic fatty liver disease [3] , [4] . Progression from chronic hepatitis to hepatocellular carcinoma is characterized by infiltration of immune cells and inflammatory cytokine production [5] . TNF-α, one of the most important proinflammatory cytokines, is produced predominantly by Kupffer cells and in part by neutrophils or hepatocytes during inflammatory responses; this cytokine is critical for maintenance of chronic inflammation [2] . The increased production of TNF-α may, in turn, augment the activation of inflammatory cells and mediate the release of inflammation factors, such as interleukin-1 (IL-1), IL-6 and intercellular adhesion molecule [6] . TNF-α has pleiotropic functions in inflammatory progression depending on cell type or biological context [7] . In certain conditions, TNF-α induces apoptosis; however, recent studies have indicated that TNF-α may promote hepatocellular carcinogenesis by activating a variety of signal pathways related to cell proliferation, differentiation and survival [8] , [9] , [10] . The mechanism of inflammation linked to TNF-α and involved in hepatocellular carcinogenesis still needs to be fully elucidated. Phosphatidylinositide 3-kinases (PI3K) are a family of enzymes involved in cellular functions such as cell growth, proliferation, differentiation, motility, survival and intracellular trafficking, which in turn are involved in cancer. Akt (now also called Akt1), a PI3K downstream target, is involved in cellular survival pathways by inhibiting apoptotic processes. PI3K/Akt can be activated in response to numerous cytokines, including TNF-α (ref. 11 ). Active Akt can protect cells from TNF-α-induced apoptosis and can facilitate cellular survival and proliferation [12] . Experimentally, Akt promotes proliferation in a variety of cell and animal models [13] . Akt is frequently induced in human HCC samples, and overexpression of Akt in mouse livers results in tumour development [14] , [15] . Disruption of the PI3K/Akt axis correlates with HCC growth arrest and/or apoptosis [16] . The mechanism of TNF-α-induced Akt activation in HCC is still unclear, and the interaction between TNF-α and Akt in HCC needs to be further investigated A family of seven-transmembrane domain G-protein-coupled receptors (GPCRs) constitutes the largest known superfamily for signal transduction and transmission [17] . GPCRs control a variety of physiological and pathological processes such as neurotransmission, pain, carcinogenesis and inflammation [18] . Both conformational change and phosphorylation increase the affinity of the receptor for a small family of multifunctional GPCR regulatory or adaptor proteins known as the β-arrestins (ARRBs), including two superfamily members β-arrestin1 (ARRB1) and β-arrestin2 (ARRB2). This association blocks subsequent G protein activation and has an important role in traditional GPCR desensitization [19] . Several members of the GPCR family, including GPCR kinase-2 (GRK2) and ARRBs, have been implicated in the TNF-α-related inflammatory reaction [20] , [21] . Hepatitis B virus (HBV) is one of the most common aetiologic factors of HCC. A high prevalence of HCC arising from the background of HBV infection suggests that HCC paracancerous is an important precancerosis [22] . To analyse the possible association of GPCR family members with hepatocarcinogenesis, we performed a gene assay to screen the expression of GPCR family genes in liver tissues, including normal liver tissues, HCC paracancerous specimens and HCC samples with HBV-induced hepatitis. We found that ARRB1 , but not ARRB2 , was clearly upregulated in hepatocellular carcinogenesis. ARRB1 was originally identified as a signal terminator for GPCR signalling, but recent findings demonstrate that ARRB1 serves as a scaffold protein and functions as a signal transducer by facilitating interaction of signalling molecules. A number of studies have investigated the role of ARRB1 in cancer, including leukaemia, colon, gastric and breast cancers [23] . ARRB1 can promote tumour angiogenesis by providing a suitable microenvironment in xenograft tumour progression [24] . ARRB1 also has been reported to play a role in cell proliferation, apoptosis and differentiation through several signal pathways [25] , [26] . Additional studies have shown that ARRB1 is involved in the activation of PI3K/Akt pathway and influences apoptosis or cell survival [23] . However, the role of ARRB1 in hepatocellular carcinogenesis remains unknown. In this study, our data show that hepatic inflammation clearly induces TNF-α production and ARRB1 expression. TNF-α directly induces hepatic ARRB1 expression and enhances ARRB1 interaction with Akt through binding to boost Akt phosphorylation and PCNA upregulation, resulting in hepatocellular malignant proliferation and carcinogenesis. Our data suggest that ARRB1 is involved in hepatocellular carcinogenesis via inflammation-mediated Akt signal, and TNF-α/ARRB1/Akt axis plays a critical role. The results indicate that ARRB1 may be a potential therapeutic target for HCC. ARRB1 is involved in hepatocellular carcinogenesis HCC is an inflammation-linked cancers in which inflammatory cells and cytokines play a critical role. In this study, a small amount of CD68 and myeloperoxidase (MPO) staining was observed, indicating minimal macrophage and neutrophil infiltration in normal liver tissues. In contrast, a large amount of CD68 and MPO was found in both paracancerous tissues and HCC samples, compared with normal liver tissues ( Fig. 1a ). The CD68 in paracancerous tissue was significantly higher than HCC, whereas the MPO in HCC was clearly higher than that in paracancerous tissue ( Fig. 1b ). The results indicated that macrophage and neutrophil infiltration was involved in hepatic carcinogenesis. Proinflammatory cytokines, including TNF-α, IL-6 and IL-1β, were markedly induced both in paracancerous tissues and hepatocellular carcinoma, and their expression in paracancerous tissues was notably higher than that in HCC ( Fig. 1c,d ). A gene expression microanalysis was performed to screen for human gene expression alteration of the GPCR family among three normal liver tissues and three pairs of HCC paracancerous tissues as well as HCC tissues, which were characterized by HBV-induced hepatitis. We found that ARRB1 , but not ARRB2 , showed a distinctly higher expression in HCC paracancerous than normal liver tissues, but no significant difference was found between HCC paracancerous tissues and HCC tissues, suggesting that ARRB1 may play a meaningful role in hepatocellular carcinogenesis ( Fig. 2a–d ). Furthermore, at both mRNA and protein levels, ARRB expression was examined in 7 normal liver tissues, 89 HCC, and their corresponding adjacent paracancerous tissues. Results showed that ARRB1 expression, but not ARRB2, was significantly upregulated in paracancerous tissues and hepatocellular carcinoma, compared with normal liver tissues ( Fig. 1e–g ). Immunohistochemistry staining was performed to confirm ARRB1 expression in 7 normal liver tissues and 89 paired HCC with adjacent paracancerous tissues. A small amount of ARRB1 expression was observed in normal liver tissues. In contrast, prominent ARRB1 staining, predominantly in cytoplasm, was found in both HCC and paracancerous tissues ( Fig. 1h ). 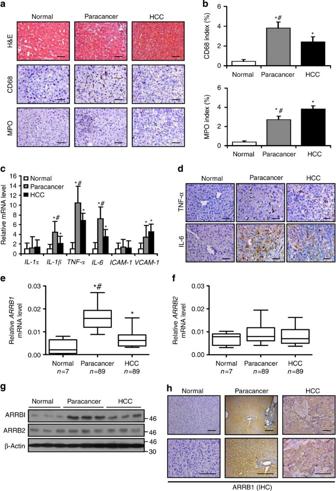Figure 1: ARRB1 is involved in inflammation-mediated hepatocellular carcinogenesis in human tissues. (a) H&E staining (top), CD68 staining for macrophages (middle) and MPO staining for neutrophils (bottom), from human normal liver tissue, hepatocellular carcinoma (HCC) and its paracancerous tissue. Scale bar, 50 μm. (b) Index of CD68 (top) and MPO (bottom) positive cells in the liver was measured by counting 1,000 cells/sample. Values are mean±s.d. (n=5 in each group), *P<0.05 compared with normal liver tissues,#P<0.05 compared with HCC using Student’st-test. (c) Expression of indicated inflammatory cytokines mRNA in human normal liver tissue, HCC and its paracancerous tissue were analysed by real-time PCR. Values are mean±s.d. (n=5 in each group), Student’st-test used: *P<0.05 compared with normal liver tissues,#P<0.05 compared with HCC. (d) Representative images of TNF-α (top) and IL-6 (bottom) immunohistochemical staining in human normal liver tissue, HCC and its paracancerous tissue. Scale bar, 50 μm. (e,f) ARRB1 and ARRB2 mRNA levels in human normal liver tissue, HCC and its paracancerous tissue were determined by real-time PCR. Values are mean±s.d. (n=7 for normal liver,n=89 for HCC and its paracancerous group respectively), *P<0.05 compared with normal liver tissues,#P<0.05 compared with HCC by using one-way ANOVA test. (g) ARRB1 and ARRB2 protein expression in human normal liver tissue, HCC and its paracancerous tissue determined by western blotting assay. (h) ARRB1 and ARRB2 protein expression in human normal liver tissue, HCC and its paracancerous tissue determined by immunohistochemical staining. Scale bar, 100 μm. Clear ARRB1 expression was observed in both HCC and paracancerous tissues, and strong positive staining of ARRB1 in the paracancerous tissues was significantly higher (78.7%) than in HCC tissues (60.7%), as shown in Supplementary Table 1 . These results demonstrated that ARRB1 is involved in inflammation-mediated hepatocellular carcinogenesis and plays a critical role in carcinogenesis. Figure 1: ARRB1 is involved in inflammation-mediated hepatocellular carcinogenesis in human tissues. ( a ) H&E staining (top), CD68 staining for macrophages (middle) and MPO staining for neutrophils (bottom), from human normal liver tissue, hepatocellular carcinoma (HCC) and its paracancerous tissue. Scale bar, 50 μm. ( b ) Index of CD68 (top) and MPO (bottom) positive cells in the liver was measured by counting 1,000 cells/sample. Values are mean±s.d. ( n =5 in each group), * P <0.05 compared with normal liver tissues, # P <0.05 compared with HCC using Student’s t -test. ( c ) Expression of indicated inflammatory cytokines mRNA in human normal liver tissue, HCC and its paracancerous tissue were analysed by real-time PCR. Values are mean±s.d. ( n =5 in each group), Student’s t -test used: * P <0.05 compared with normal liver tissues, # P <0.05 compared with HCC. ( d ) Representative images of TNF-α (top) and IL-6 (bottom) immunohistochemical staining in human normal liver tissue, HCC and its paracancerous tissue. Scale bar, 50 μm. ( e , f ) ARRB1 and ARRB2 mRNA levels in human normal liver tissue, HCC and its paracancerous tissue were determined by real-time PCR. Values are mean±s.d. ( n =7 for normal liver, n =89 for HCC and its paracancerous group respectively), * P <0.05 compared with normal liver tissues, # P <0.05 compared with HCC by using one-way ANOVA test. ( g ) ARRB1 and ARRB2 protein expression in human normal liver tissue, HCC and its paracancerous tissue determined by western blotting assay. ( h ) ARRB1 and ARRB2 protein expression in human normal liver tissue, HCC and its paracancerous tissue determined by immunohistochemical staining. Scale bar, 100 μm. 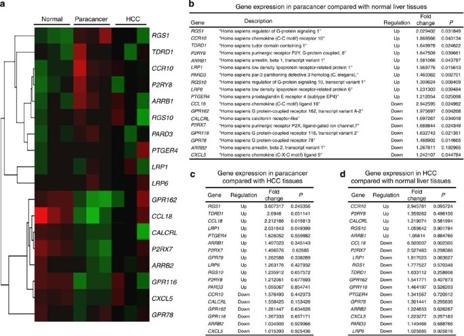Figure 2: GPCR-related proteins involved in inflammation-mediated human HCC. (a) Two-dimensional hierarchical clustering results for GPCR relative genes among normal liver tissue, HCC and its paracancerous tissues. The fold changes in mRNA levels in paracancerous tissues and HCC relative to normal liver tissues are represented by green and red squares, showing decreased and increased levels, respectively. (b,c) GPCR relative gene expression in paracancerous tissue compared with normal liver and HCC tissues. The ratio represents the expression value in paracancerous tissue compared with the expression level in normal liver and HCC tissues. (d) GPCR relative gene expression in HCC tissue compared with normal liver tissue.P<0.05 by using Student’st-test. Full size image Figure 2: GPCR-related proteins involved in inflammation-mediated human HCC. ( a ) Two-dimensional hierarchical clustering results for GPCR relative genes among normal liver tissue, HCC and its paracancerous tissues. The fold changes in mRNA levels in paracancerous tissues and HCC relative to normal liver tissues are represented by green and red squares, showing decreased and increased levels, respectively. ( b , c ) GPCR relative gene expression in paracancerous tissue compared with normal liver and HCC tissues. The ratio represents the expression value in paracancerous tissue compared with the expression level in normal liver and HCC tissues. ( d ) GPCR relative gene expression in HCC tissue compared with normal liver tissue. P <0.05 by using Student’s t -test. Full size image Inflammation induces hepatocellular ARRB1 expression in mice Our data showed that ARRB1 was significantly upregulated in HCC and adjacent paracancerous tissues in infected HBV patients. However, it remained unknown whether ARRB1 expression was directly induced by inflammation in animals. We established two mouse hepatitis models by tetrachloromethane (CCl 4 , a well-known hepatotoxin) or diethylnitrosamine (DEN, a genotoxic drug that induces hepatocellular carcinogenesis). After CCl 4 or DEN treatment, the hepatic inflammatory mediators, including IL-1α , IL-1β , IL-6 , TNF-α , ICAM-1 and VCAM-1 , were markedly upregulated ( Fig. 3a,b ). Simultaneously, western blotting showed that the protein levels of TNF-α and ARRB1 were markedly induced in hepatic tissues after CCl 4 treatment ( Fig. 3c,d ) or DEN treatment ( Fig. 3e,f ). Furthermore, immunohistochemistry staining confirmed that the expression of TNF-α and ARRB1 was clearly increased in hepatocytes after CCl 4 treatment or DEN treatment ( Fig. 3g,h ). The data indicated that the CCl 4 - or DEN-induced inflammatory response significantly enhances hepatocellular ARRB1 expression in mice. 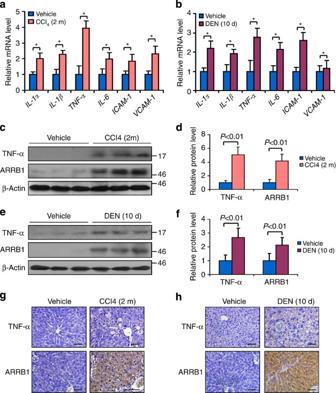Figure 3: Inflammation induced hepatocellular ARRB1 expression in mice. (a) Expression of indicated inflammatory mediators mRNA in the mice livers after either physiological saline (Vehicle) or CCl4 (15 mg kg−1) intraperitoneal injection twice a week for 2 months were analysed by real-time PCR. Values are mean±s.d. (n=6 in each group), *P<0.05 compared with vehicle treatment by using Student’st-test. (b) mRNA expression of inflammatory mediators in the mouse livers after either physiological saline (Vehicle) or 100 mg kg−1of DEN intraperitoneal injection for 10 days were analysed by real-time PCR. Values are mean±s.d. (n=6 in each group), Student’st-test used: *P<0.05 compared with vehicle treatment. (c,d) Protein expression of TNF-α and ARRB1 in the livers of WT mice was determined by western blotting after either physiological saline (Vehicle) or 15 mg kg−1of CCl4intraperitoneal injection twice a week for 2 months. Values are mean±s.d. (n=6 in each group).P<0.01 by using Student’st-test. (e,f) Protein expression of TNF-α and ARRB1 in the livers of WT mice was determined by western blotting 10 days after either physiological saline (Vehicle) or 100 mg kg−1of DEN intraperitoneal injection. Values are mean±s.d. (n=6 in each group).P<0.05 using Student’st-test. (g,h) Representative images of TNF-α (top) and IL-6 (bottom) staining in CCL4-induced liver cirrhosis and DEN-induced liver inflammation. Scale bar, 50 μm. Figure 3: Inflammation induced hepatocellular ARRB1 expression in mice. ( a ) Expression of indicated inflammatory mediators mRNA in the mice livers after either physiological saline (Vehicle) or CCl4 (15 mg kg −1 ) intraperitoneal injection twice a week for 2 months were analysed by real-time PCR. Values are mean±s.d. ( n =6 in each group), * P <0.05 compared with vehicle treatment by using Student’s t -test. ( b ) mRNA expression of inflammatory mediators in the mouse livers after either physiological saline (Vehicle) or 100 mg kg −1 of DEN intraperitoneal injection for 10 days were analysed by real-time PCR. Values are mean±s.d. ( n =6 in each group), Student’s t -test used: * P <0.05 compared with vehicle treatment. ( c , d ) Protein expression of TNF-α and ARRB1 in the livers of WT mice was determined by western blotting after either physiological saline (Vehicle) or 15 mg kg −1 of CCl 4 intraperitoneal injection twice a week for 2 months. Values are mean±s.d. ( n =6 in each group). P <0.01 by using Student’s t -test. ( e , f ) Protein expression of TNF-α and ARRB1 in the livers of WT mice was determined by western blotting 10 days after either physiological saline (Vehicle) or 100 mg kg −1 of DEN intraperitoneal injection. Values are mean±s.d. ( n =6 in each group). P <0.05 using Student’s t -test. ( g , h ) Representative images of TNF-α (top) and IL-6 (bottom) staining in CCL 4 -induced liver cirrhosis and DEN-induced liver inflammation. Scale bar, 50 μm. Full size image ARRB1 deficiency suppresses hepatocellular carcinogenesis The preceding data have shown that the inflammatory response induces hepatocellular ARRB1 expression and that ARRB1 may be involved in inflammation-mediated hepatocellular carcinogenesis. To confirm whether ARRB1 plays a role in inflammation-mediated hepatocellular carcinogenesis, we induced hepatocarcinogenesis with the inflammatory genotoxic drug DEN in ARRB1 -deficient mice. Male mice were treated with a single injection of DEN at age 15 days, and they efficiently developed HCC. Tumour incidence and tumour weight as well as tumour size were evaluated 9 months after DEN treatment. Tumours developed in all mice after 9 months; however, the hepatocarcinogenesis was significantly reduced in ARRB1 -knockout (KO) mice compared with ARRB1 wild type (WT) ( Fig. 4a,b ). The relative liver weight versus body weight in ARRB1 -KO mice was reduced by 2.5-fold compared with WT mice (1.7±1.2 versus 4.6±1.1%), as shown in Fig. 4c . The tumour incidence in ARRB1 -KO mice was decreased approximately threefold compared with WT mice (3.2±1.7 versus 9.6±2.4) ( Fig. 4d ). The maximal tumour size and average tumour size also were markedly decreased in ARRB1 -KO mice compared with those in WT mice ( Fig. 4e,f ). Tumour samples were confirmed by histopathological analysis to be hepatocellular cancer ( Fig. 4g ). Next, we analysed tumour cell proliferation by Ki67 immunohistochemistry staining. The results showed that the malignant cell proliferation was significantly repressed and that the numbers of Ki67-positive cells were reduced by ∼ 48% in ARRB1- KO mice compared with ARRB1 WT mice ( Fig. 4h,i ). Simultaneously, the effect of ARRB2 deficiency in DEN-induced hepatocellular carcinogenesis was also investigated, and the results showed that ARRB2 deficiency did not affect hepatocellular cancer initiation and development ( Supplementary Fig. 1 ). Furthermore, a tumorigenicity experiment in Balb/c nude mice showed that ARRB1, but not ARRB2, significantly promoted xenograft tumour growth in vivo ( Fig. 5 ). These results suggest that deficiency of ARRB1, but not ARRB2, suppresses DEN-induced hepatocellular carcinogenesis by downregulating hepatocellular proliferation. 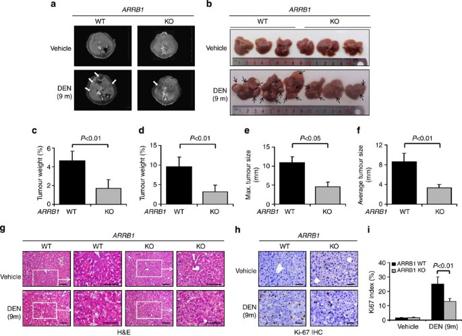Figure 4: ARRB1 deficiency suppressed DEN-induced hepatocellular carcinogenesis. WT andARRB1-KO mice were treated with a single DEN (15 mg kg−1) intraperitoneal injection, and livers were harvested at 9 months. (a) MRI images of DEN-induced liver tumours after gadobenate dimeglumine injection (0.1 mmol kg−1). (b) Photographs of DEN-induced liver tumours at 9 months. (c) Quantification of liver average weight as a percentage of body weight (n=10 in each group). (d) Average numbers of liver tumours in WT andARRB1-KO mice at 9 months (n=10 in each group). (e) Maximal tumour size measured by caliper (n=10 in each group). (f) Average liver tumour diameter by caliper (n=10 in each group). (g) Representative H&E staining of DEN-induced liver tumours in WT andARRB1KO mice. Scale bar, 100 μm. (h,i) Ki67 staining in DEN-induced liver tumours at 9 months after DEN injection (Scale bar, 50 μm) and the Ki67 index was scored (n=6 in each group). All values are mean±s.d.P<0.01 orP<0.05 by using Student’st-test. Figure 4: ARRB1 deficiency suppressed DEN-induced hepatocellular carcinogenesis. WT and ARRB1 -KO mice were treated with a single DEN (15 mg kg −1 ) intraperitoneal injection, and livers were harvested at 9 months. ( a ) MRI images of DEN-induced liver tumours after gadobenate dimeglumine injection (0.1 mmol kg −1 ). ( b ) Photographs of DEN-induced liver tumours at 9 months. ( c ) Quantification of liver average weight as a percentage of body weight ( n =10 in each group). ( d ) Average numbers of liver tumours in WT and ARRB1 -KO mice at 9 months ( n =10 in each group). ( e ) Maximal tumour size measured by caliper ( n =10 in each group). ( f ) Average liver tumour diameter by caliper ( n =10 in each group). ( g ) Representative H&E staining of DEN-induced liver tumours in WT and ARRB1 KO mice. Scale bar, 100 μm. ( h , i ) Ki67 staining in DEN-induced liver tumours at 9 months after DEN injection (Scale bar, 50 μm) and the Ki67 index was scored ( n =6 in each group). All values are mean±s.d. P <0.01 or P <0.05 by using Student’s t -test. 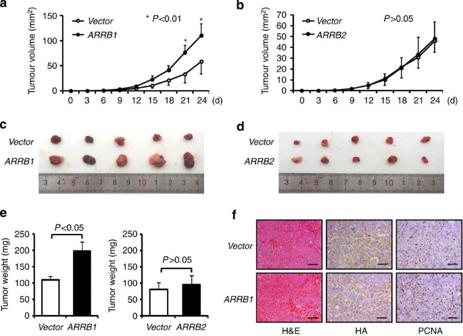Figure 5:ARRB1upregulated the growth of xenograft HCC. (a) The growth curve of xenograft tumour of Hep3B cells subjected toARRB1-HAorvector-HAtransfection. Data were expressed as mean±s.d. (n=5 in each group), *P<0.05 by using Student’st-test. (b) The growth curve of xenograft tumours of Hep3B cells subjected toARRB2-HAtransfection orvector-HAtransfection. Data were expressed as mean±s.d. (n=5 in each group). (c) Xenograft tumours from Hep3B cells subjected toARRB1-HAtransfection (bottom) or vector-HAtransfection (top) at the end of the experiment. (d) Xenograft tumours from Hep3B cells subjected toARRB2-HAtransfection (bottom) or vector-HAtransfection (top) at the end of the experiment. (e) Xenograft tumour weights from different treatment groups at the end of the experiment. Data were expressed as mean±s.d. (n=5 in each group). (f) Representative H&E, HA and PCNA staining from xenograft tumours in Hep3B cells subjected to ARRB1-HA or vector-HA transfection. Scale bar, 100 μm.P<0.05 using Student’st-test. Full size image Figure 5: ARRB1 upregulated the growth of xenograft HCC. ( a ) The growth curve of xenograft tumour of Hep3B cells subjected to ARRB1-HA or vector-HA transfection. Data were expressed as mean±s.d. ( n =5 in each group), * P <0.05 by using Student’s t -test. ( b ) The growth curve of xenograft tumours of Hep3B cells subjected to ARRB2-HA transfection or vector-HA transfection. Data were expressed as mean±s.d. ( n =5 in each group). ( c ) Xenograft tumours from Hep3B cells subjected to ARRB1-HA transfection (bottom) or vector -HA transfection (top) at the end of the experiment. ( d ) Xenograft tumours from Hep3B cells subjected to ARRB2-HA transfection (bottom) or vector -HA transfection (top) at the end of the experiment. ( e ) Xenograft tumour weights from different treatment groups at the end of the experiment. Data were expressed as mean±s.d. ( n =5 in each group). ( f ) Representative H&E, HA and PCNA staining from xenograft tumours in Hep3B cells subjected to ARRB1-HA or vector-HA transfection. Scale bar, 100 μm. P <0.05 using Student’s t -test. Full size image Deleted ARRB1 inhibits hepatic compensatory proliferation The preceding data demonstrated that ARRB1 is a potent mediator of HCC progression, and previous studies suggested that compensatory proliferation after extensive hepatocyte apoptosis induced by DEN is essential for DEN-induced HCC development [27] . To investigate the mechanism of ARRB1 in hepatocellular carcinogenesis, we next analysed whether ARRB1 enhanced compensatory hepatocyte proliferation to contribute to hepatocellular carcinogenesis by inhibiting apoptosis in DEN-treated mice. Induction of hepatic MPO activity, which is an indicator of neutrophil infiltration, showed no significant difference between ARRB1 WT mice and ARRB1 -KO mice 10 days after DEN treatment ( Fig. 6a ). Histopathological analysis showed significant hepatocyte death with inflammatory cell infiltration in DEN-treated mice ( Fig. 6b ). Surprisingly, DEN-induced apoptosis was markedly increased in ARRB1- KO mice, and the increase was ∼ 50% greater than in ARRB1 WT mice ( Fig. 6c,d ). Furthermore, hepatic active caspase-3 was assessed by western blotting and immunohistochemistry staining, which showed that DEN distinctly induced caspase-3 activation and that active caspase-3 was visibly upregulated in ARRB1- KO mice compared with ARRB1 WT mice ( Fig. 6e–g ). Moreover, hepatocellular compensatory proliferation was also significantly upregulated in DEN-treated mice; however, the compensatory proliferation was clearly repressed in ARRB1 KO compared with ARRB1 WT mice ( Fig. 6h–j ). These results demonstrated that ARRB1 inhibits inflammation-induced hepatocellular apoptosis and enhances hepatocellular compensatory proliferation in DEN-treated mice. 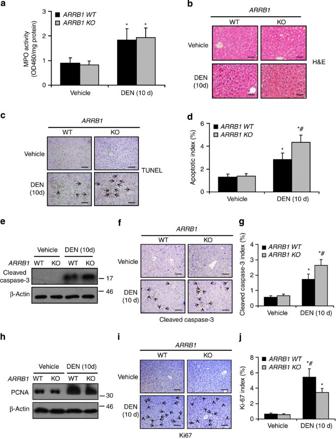Figure 6: Effects ofARRB1deletion on inflammation-induced hepatocellular apoptosis and hepatocellular proliferation. (a) MPO activity was determined in DEN-treated WT andARRB1-KO mice. Values are mean±s.d. (n=6 in each group), Student’st-test used: *P<0.05 compared with vehicle treatment. (b) Representative H&E staining images of liver tissues at 10 days after DEN injection in WT andARRB1-KO mice. Scale bar, 50 μm. (c,d) Liver tissues were harvested from WT andARRB1-KO mice at 0 and 10 days after injection of DEN (100 mg kg−1). TUNEL (brown) was stained in the liver (Scale bar, 100 μm), and the apoptotic index was measured by counting TUNEL signals. TUNEL index was measured. Values are mean±s.d. (n=6 in each group), *P<0.05 compared with vehicle treatment,#P<0.05 compared with WT mice by using Student’st-test. (e) Cleaved caspase-3 protein expression was determined by western blotting. (f,g) Cleaved caspase-3 (brown) was stained in liver tissues (Scale bar, 100 μm), and the cleaved caspase-3 index was detected. Values are mean±s.d. (n=6 in each group), *P<0.05 compared with vehicle treatment,#P<0.05 compared with WT mice using Student’st-test. (h) PCNA level in the livers was determined by western blotting. (i,j) Ki-67 expression (brown) was checked by immunohistochemical staining (Scale bar, 100 μm), and the Ki67 index was measured by counting Ki-67 signals. Values are mean±s.d. (n=6 in each group), Student’st-test used: *P<0.05 compared with vehicle treatment,#P<0.05 compared with ARRB1-KO mice. Figure 6: Effects of ARRB1 deletion on inflammation-induced hepatocellular apoptosis and hepatocellular proliferation. ( a ) MPO activity was determined in DEN-treated WT and ARRB1- KO mice. Values are mean±s.d. ( n =6 in each group), Student’s t -test used: * P <0.05 compared with vehicle treatment. ( b ) Representative H&E staining images of liver tissues at 10 days after DEN injection in WT and ARRB1- KO mice. Scale bar, 50 μm. ( c , d ) Liver tissues were harvested from WT and ARRB1- KO mice at 0 and 10 days after injection of DEN (100 mg kg −1 ). TUNEL (brown) was stained in the liver (Scale bar, 100 μm), and the apoptotic index was measured by counting TUNEL signals. TUNEL index was measured. Values are mean±s.d. ( n =6 in each group), * P <0.05 compared with vehicle treatment, # P <0.05 compared with WT mice by using Student’s t -test. ( e ) Cleaved caspase-3 protein expression was determined by western blotting. ( f , g ) Cleaved caspase-3 (brown) was stained in liver tissues (Scale bar, 100 μm), and the cleaved caspase-3 index was detected. Values are mean±s.d. ( n =6 in each group), * P <0.05 compared with vehicle treatment, # P <0.05 compared with WT mice using Student’s t -test. ( h ) PCNA level in the livers was determined by western blotting. ( i , j ) Ki-67 expression (brown) was checked by immunohistochemical staining (Scale bar, 100 μm), and the Ki67 index was measured by counting Ki-67 signals. Values are mean±s.d. ( n =6 in each group), Student’s t -test used: * P <0.05 compared with vehicle treatment, # P <0.05 compared with ARRB1-KO mice. Full size image Proinflammatory factor TNF-α facilitates ARRB1 expression The proinflammatory factor TNF-α plays a pivotal role in inflammatory responses, and it is one of the most important inflammatory factors closely related with GPCRs. It is unclear whether TNF-α facilitates hepatic ARRB1 expression. First, we treated the HCC cell line HepG2 and an immortal human liver cell line LO2 with TNF-α, and we observed that TNF-α significantly induced ARRB1 expression ( Fig. 7a,b ). Then, we treated ARRB1 WT mice by TNF-α intraperitoneal injection, and we also found that TNF-α remarkably induced hepatic ARRB1 expression; ARRB1 mRNA was increased ∼ 2.6-fold at 2 h after TNF-α treatment compared with vehicle-treated mice, and ARRB1 protein was also significantly upregulated at 6 h after TNF-α treatment compared with vehicle-treated mice ( Fig. 7c,d ). Our data showed that TNF-α upregulated ARRB1 expression in human HepG2 and LO2 cell lines in a dose-dependent and time-dependent manner and that TNF-α also induced hepatic ARRB1 expression in mice. The data indicated that the proinflammatory mediator TNF-α facilitates ARRB1 expression in vitro and in vivo . 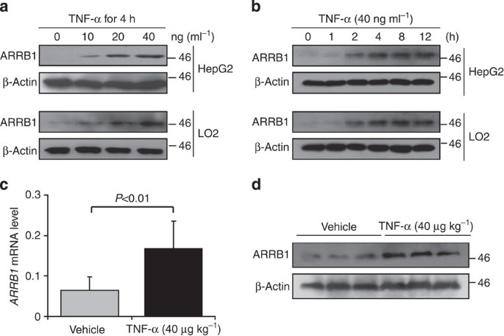Figure 7: Proinflammatory mediator TNF- α enhanced ARRB1 expression. (a,b) HepG2 and LO2 cells were treated with TNF-α, and expression of ARRB1 was analysed by western blotting. Shown is a representative result of three experiments. (c,d) WT mice were treated by TNF-α (40 μg kg−1) intraperitoneal injection for 4 h, and hepatic expression ofARRB1mRNA and ARRB1 protein were analysed by real-time PCR and western blotting, respectively. Values are mean±s.d. (n=6 in each group).P<0.01 by using Student’st-test. Figure 7: Proinflammatory mediator TNF- α enhanced ARRB1 expression. ( a , b ) HepG2 and LO2 cells were treated with TNF-α, and expression of ARRB1 was analysed by western blotting. Shown is a representative result of three experiments. ( c , d ) WT mice were treated by TNF-α (40 μg kg −1 ) intraperitoneal injection for 4 h, and hepatic expression of ARRB1 mRNA and ARRB1 protein were analysed by real-time PCR and western blotting, respectively. Values are mean±s.d. ( n =6 in each group). P <0.01 by using Student’s t -test. Full size image ARRB1 promotes hepatocellular proliferation via Akt pathway The PI3K/Akt signalling pathway is related to HCC cell proliferation [16] . Previous reports have shown that ARRB1 mediates Akt phosphorylation to activate PI3K/Akt signalling in response to a variety of stimuli [28] . ARRB1 mRNA expression levels in HepG2, Hep3B, Huh7 and LO2 cell lines were analysed by real-time PCR. The data showed that among these four cell lines, HepG2 and LO2 had mild ARRB1 mRNA expression, Huh7 had strong expression, and Hep3B had low ARRB1 mRNA expression ( Supplementary Fig. 2 ). Therefore, we transfected ARRB1 plasmid into HepG2 and LO2 cell lines, and we found that cell viability was significantly increased, Akt was markedly phosphorylated, and PCNA expression was markedly induced ( Fig. 8a–c ). Then, we downregulated ARRB1 by siRNA in HepG2 and LO2 cell lines and observed that cell viability was significantly reduced, Akt phosphorylation was markedly restrained and PCNA expression was clearly inhibited ( Fig. 8d–f ). Furthermore, we inhibited Akt activity by the Akt inhibitor A6730 in HepG2 and LO2 cell lines and found that cell viability was significantly reduced, Akt phosphorylation was fully restrained, and PCNA expression was markedly inhibited ( Supplementary Fig. 3a–c ). Simultaneously, we induced ARRB1 expression by TNF-α in HepG2 and LO2 cell lines and found that Akt inhibitor A6730-treatment significantly reduced cell viability, fully reduced Akt phosphorylation, and markedly inhibited PCNA expression ( Supplementary Fig. 3d–f ). Next, we treated HepG2 and LO2 cell lines with A6730 after ARRB1 plasmid transfection and also found that cell viability was significantly downregulated, Akt phosphorylation was fully restrained and PCNA expression was markedly reduced ( Fig. 8g–i ). Sequentially, we overexpressed ARRB1 to examine the effect of ARRB1 on cell proliferation by ARRB1 plasmid transfection in HepG2 and Hep3B as well as LO2 cell lines, and we observed that ARRB1 significantly promoted hepatocellular growth and colony formation among three cell lines ( Fig. 9 ). Furthermore, downregulation of ARRB1 expression in HepG2, Huh7 and LO2 by siRNA inhibited hepatocellular proliferation in vitro ( Supplementary Fig. 4 ). Altogether, these results suggest that ARRB1 promotes hepatocellular proliferation through PI3K/Akt signalling. 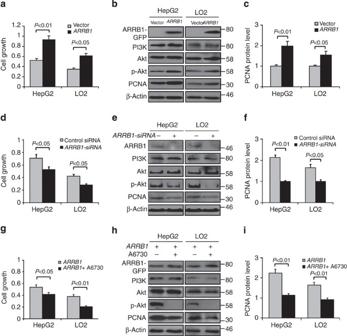Figure 8: ARRB1 promoted hepatocellular proliferation through PI3K/Akt signalling. (a–c)ARRB1transfection significantly increased cell growth, enhanced Akt phosphorylation and PCNA overexpression. The experiment was repeated three times. (d–f)ARRB1expression was silenced byARRB1-siRNA. ARRB1 knockdown significantly restrained cell growth, reduced Akt phosphorylation and PCNA product in HepG2 and LO2 cell lines. (g–i) Cells were treated by Akt inhibitor afterARRB1transfection. Akt inhibitor clearly inhibited ARRB1-induced cell growth and Akt phosphorylation, and repressed PCNA expression. All values are the means±s.d. in three separate experiments and repeated three times.P<0.01 orP<0.05 using Student’st-test. Figure 8: ARRB1 promoted hepatocellular proliferation through PI3K/Akt signalling. ( a – c ) ARRB1 transfection significantly increased cell growth, enhanced Akt phosphorylation and PCNA overexpression. The experiment was repeated three times. ( d – f ) ARRB1 expression was silenced by ARRB1 -siRNA. ARRB1 knockdown significantly restrained cell growth, reduced Akt phosphorylation and PCNA product in HepG2 and LO2 cell lines. ( g – i ) Cells were treated by Akt inhibitor after ARRB1 transfection. Akt inhibitor clearly inhibited ARRB1-induced cell growth and Akt phosphorylation, and repressed PCNA expression. All values are the means±s.d. in three separate experiments and repeated three times. P <0.01 or P <0.05 using Student’s t -test. 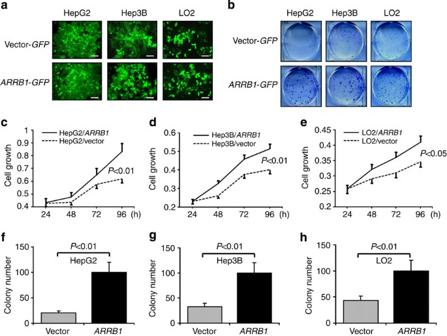Figure 9: ARRB1 promoted hepatocellular proliferationin vitro. Cells were stably transfected with pcDNA3.0/ARRB1-GFPor pcDNA3.0/GFP(Vector) to overexpress ARRB1 in HepG2 and Hep3B as well as LO2 cell lines. (a) Cells stably expressed ARBB1 after pcDNA3.0/ARRB1-GFPtransfection for 48 h. Scale bar, 50 μm. (b) Colonies were formed in pcDNA3.0/ARRB1-GFPtransfected cells after G418 selection. (c–e) Cell growth curve after pcDNA3.0/ARRB1-GFPtransfection. (f–h) Quantitation of colony formation in pcDNA3.0/ARRB1-GFPtransfected cells after G418 selection. All values are the means±s.d. in three separate experiments and repeated three times.P<0.01 orP<0.05 using Student’st-test. Full size image Figure 9: ARRB1 promoted hepatocellular proliferation in vitro . Cells were stably transfected with pcDNA3.0/ ARRB1-GFP or pcDNA3.0/ GFP (Vector) to overexpress ARRB1 in HepG2 and Hep3B as well as LO2 cell lines. ( a ) Cells stably expressed ARBB1 after pcDNA3.0/ ARRB1-GFP transfection for 48 h. Scale bar, 50 μm. ( b ) Colonies were formed in pcDNA3.0/ ARRB1-GFP transfected cells after G418 selection. ( c – e ) Cell growth curve after pcDNA3.0/ ARRB1-GFP transfection. ( f – h ) Quantitation of colony formation in pcDNA3.0/ ARRB1-GFP transfected cells after G418 selection. All values are the means±s.d. in three separate experiments and repeated three times. P <0.01 or P <0.05 using Student’s t -test. Full size image Inflammation-induced HCC depends on ARRB1/Akt activation Although the preceding results have demonstrated that ARRB1 mediates Akt phosphorylation in vitro , it was unclear whether ARRB1 mediates Akt phosphorylation in DEN-induced hepatocellular carcinogenesis. We examined hepatic Akt phosphorylation in DEN-treated mice to investigate the effect of ARRB1 on Akt phosphorylation in response to hepatocyte survival and proliferation using ARRB1 -KO and ARRB1 WT mice. Although ARRB1 deficiency did not affect TNF-α expression, it significantly attenuated DEN-induced Akt activation and PCNA expression ( Fig. 10a , Supplementary Fig. 5a ). In DEN-induced hepatocellular carcinogenesis, PI3K and Akt expression were markedly increased, Akt phosphorylation was remarkably upregulated and PCNA expression was clearly enhanced in HCC tissues compared with paracancerous tissues ( Fig. 10b ). Although ARRB1 deficiency did not depress PI3K and Akt expression, it clearly repressed Akt phosphorylation and PCNA expression, and immunofluorescence staining showed that Akt activation was distinctly inhibited in both HCC tissues and paracancerous tissues ( Fig. 10b , Supplementary Fig. 5b–d ). Furthermore, ARRB1 expression also correlated with Akt activity in human HCC tissue samples ( Supplementary Fig. 6a–c ). In addition, we tested the effect of TNF-α on Akt phosphorylation using ARRB1 WT mice and found that ARRB1 expression and Akt phosphorylation were significantly upregulated 6 h after intraperitoneal TNF-α injection ( Fig. 10c ). However, pretreatment with Akt inhibitor A6730 in mice markedly depressed hepatic Akt phosphorylation, but not ARRB1 expression ( Fig. 10d ). The preceding data showed that ARRB1 enhanced Akt phosphorylation. However, whether the effect of ARRB1 is mediated by interacting with Akt was unclear. To confirm this mechanism, the interaction between ARRB1 and Akt in mammalian cells was analysed by co-immunoprecipitation. The interaction between ARRB1 and Akt was examined in HepG2 cells by co-immunoprecipitation after ARRB1 transfection, and the results showed that ARRB1 interacted with Akt by binding ( Fig. 10e ). Furthermore, TNF-α notably enhanced ARRB1 expression and promoted ARRB1 interaction with Akt by binding to boost Akt phosphorylation ( Fig. 10f ). These results indicated that inflammation-induced hepatocellular malignant proliferation depends on ARRB1-mediated Akt activation, resulting in hepatocellular carcinogenesis. 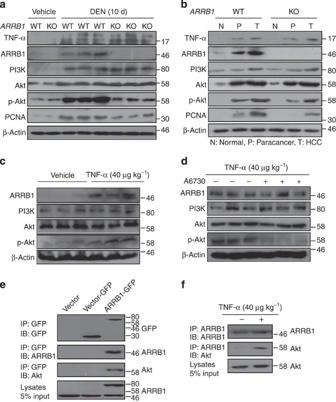Figure 10: Inflammation-induced hepatocellular carcinogenesis depended on ARRB1-mediated Akt activation. (a) DEN-induced inflammation upregulated expression of TNF-α, ARRB1, p-Akt and PCNA in mice liver, andARRB1knockout significantly inhibited the expression. (b) PI3K and Akt were markedly upregulated in DEN-induced hepatocellular carcinogenesis; however,ARRB1knockout clearly restrained Akt phosphorylation and reduced PCNA production in hepatocellular carcinogenesis. (c,d) The expression of ARRB1, PI3K, p-Akt and PCNA was analysed by western blotting in mouse livers 6 h after intraperitoneal TNF-α injection. TNF-α induced ARRB1 increase and Akt phosphorylation; however, Akt inhibitor A6730 (50 mg kg−1) pretreatment significantly repressed the Akt phosphorylation, but did not affect ARRB1 expression. (e) HepG2 cells were transfected withGFP-ARRB1as indicated. The cellular lysates were subjected to immunoprecipitation with an anti-GFP antibody. Co-immunoprecipitated endogenous Akt was detected with an anti-Akt antibody. (f) The HepG2 cells were challenged with TNF-α (40 ng ml−1) for 4 h, and then the cells were subjected to immunoprecipitation with an anti-ARRB1 antibody. Co-immunoprecipitated endogenous Akt was detected with an anti-Akt antibody. Shown is a representative result of three experiments. IP=immunoprecipitate; IB=immunoblot. Figure 10: Inflammation-induced hepatocellular carcinogenesis depended on ARRB1-mediated Akt activation. ( a ) DEN-induced inflammation upregulated expression of TNF-α, ARRB1, p-Akt and PCNA in mice liver, and ARRB1 knockout significantly inhibited the expression. ( b ) PI3K and Akt were markedly upregulated in DEN-induced hepatocellular carcinogenesis; however, ARRB1 knockout clearly restrained Akt phosphorylation and reduced PCNA production in hepatocellular carcinogenesis. ( c , d ) The expression of ARRB1, PI3K, p-Akt and PCNA was analysed by western blotting in mouse livers 6 h after intraperitoneal TNF-α injection. TNF-α induced ARRB1 increase and Akt phosphorylation; however, Akt inhibitor A6730 (50 mg kg −1 ) pretreatment significantly repressed the Akt phosphorylation, but did not affect ARRB1 expression. ( e ) HepG2 cells were transfected with GFP-ARRB1 as indicated. The cellular lysates were subjected to immunoprecipitation with an anti-GFP antibody. Co-immunoprecipitated endogenous Akt was detected with an anti-Akt antibody. ( f ) The HepG2 cells were challenged with TNF-α (40 ng ml −1 ) for 4 h, and then the cells were subjected to immunoprecipitation with an anti-ARRB1 antibody. Co-immunoprecipitated endogenous Akt was detected with an anti-Akt antibody. Shown is a representative result of three experiments. IP=immunoprecipitate; IB=immunoblot. Full size image Elucidating the mechanisms related to inflammation-induced HCC has long been considered a key for unravelling critical pathways in hepatocarcinogenesis. Our data showed that the inflammation induced inflammatory mediators including TNF-α, that TNF-α enhanced ARRB1 expression, and that ARRB1 activated PI3K/Akt signalling through Akt phosphorylation, resulting in inhibition of hepatocellular apoptosis and upregulation of hepatocellular compensatory proliferation to drive hepatocyte carcinogenesis. The results demonstrated that inflammation-induced hepatocellular carcinogenesis works through the TNF-α/ARRB1/Akt axis and that ARRB1 is an essential tumour promoter in the liver. Many studies have analysed the critical role of inflammation in HCC [2] . TNF-α is one of the most important proinflammatory factors with numerous biological properties, such as apoptosis, proliferation and differentiation, and it contributes to carcinogenesis in various inflammatory conditions such as chronic viral hepatitis as well as alcoholic and non-alcoholic fatty liver diseases [29] , [30] , [31] . Administration of DEN or CCl 4 to mice induces liver injury following hepatitis [6] , [27] . Experimentally, in DEN- or CCl 4 -induced mouse hepatitis models, inflammation enhances TNF-α to promote liver tumorigenesis [32] . Targets of TNF-α downstream that execute the oncogenic functions have not been fully elucidated. GPCRs have been implicated in TNF-α-induced inflammatory responses. A gene expression assay was performed to screen for alterative GPCR relative genes among normal liver tissues, HCC tissues and its paracancerous tissues with hepatitis. The data showed that several GPCR relative genes, including ARRB1 , CCR10 , P2RY8 and RGS10 , were upregulated in HCC tissues and paracancerous tissues compared with normal liver tissues ( Fig. 2 ). P2RY8 , CCR10 and RGS10 , which were elevated in HCC tissues and their pair paracancerous tissues, have been reported to play roles in carcinoma [33] , [34] , [35] . Our data showed that ARRB1 was upregulated in human HCC tissues and its paracancerous tissues compared with normal liver tissues, but there was no significant difference between HCC tissues and paracancerous tissues, suggesting that ARRB1 may play an important role in hepatocellular carcinogenesis. ARRB1 contributes to cell proliferation, apoptosis and differentiation via signal pathways and is involved in leukaemia, colon, gastric and breast cancers [25] , [26] , [36] . Upregulation of ARRB1 in hepatitis-mediated HCC tissues and its paracancerous tissues indicated that ARRB1 is involved in inflammation-induced hepatocellular carcinogenesis. ARRB1 expression at the both mRNA and protein levels were markedly increased in human HCC tissues and paired paracancerous tissues. Inflammatory cell infiltration and inflammatory cytokine upregulation, especially TNF-α, were also observed ( Fig. 1 ). Treatment with DEN or CCl 4 significantly induced hepatic ARRB1 expression in mice; however, ARRB1 deficiency did not depress the inflammatory response ( Figs 3 and 6a ). The results indicated that ARRB1 is induced by inflammation, at least partly in connection with TNF-α, and that ARRB1 is a downstream target in inflammatory response. ARRB1 was significantly upregulated in hepatitis-mediated human HCC samples and DEN-induced mice HCC models, indicating that ARRB1 plays a critical role in inflammation-induced hepatocellular carcinogenesis. To confirm the effect of ARRB1 in inflammation-induced hepatocellular carcinogenesis, we induced hepatocarcinogenesis using DEN in ARRB1 −/− mice. The results showed that tumour number decreased by 67% and tumour load decreased by 63% in ARRB1 −/− mice compared with ARRB1 +/+ mice 9 months after DEN treatment ( Fig. 4 ). Conversely, the hepatocarcinogenesis did not show any difference in ARRB2 −/− mice compared with ARRB2 +/+ mice 9 months after DEN treatment ( Supplementary Fig. 1 ). Furthermore, a tumorigenicity experiment in nude mice showed that ARRB1, but not ARRB2, played a pivotal role in promoting xenograft tumour growth in vivo ( Fig. 5 ). These data suggest that ARRB1, but not ARRB2, plays an essential role in inflammation-induced hepatocellular carcinogenesis. It was reported that ARRB2, but not ARRB1 , is essential for the initiation and growth of intestinal tumours [37] . Thus far, ARRB1 and ARRB2 have been found to have different effects in initiation and development of malignant tumours [23] . For example, one study showed that ARRB1, but not ARRB2, was required for changes in cell morphology and ablation of tight junctions consistent with epithelial-mesenchymal transition in non-small cell lung cancer [38] . Our study also showed that ARRB1, but not ARRB2, played a crucial role in hepatocarcinogenesis. This discrepancy between ARRB1 and ARRB2 may be due to different functions between ARRB1 and ARRB2 in cellular physiology and pathophysiology. Certain studies suggest that apoptosis drives a compensatory proliferation to facilitate hepatocellular carcinogenesis in DEN-induced mice [27] . However, our study showed that lack of ARRB1 increased DEN-induced hepatocellular apoptosis, depressed hepatocellular proliferation and resulted in downregulation of hepatocellular carcinogenesis ( Fig. 6 ). The results indicate that ARRB1 is essential for HCC initiation and development by inhibiting apoptosis and promoting compensatory proliferation. The putative oncogenic function of ARRB1 in HCC was further confirmed in vitro . Overexpression of ARRB1 in hepatic cell lines (HepG2, Hep3B and LO2) significantly promoted cellular viability and colony formation ( Fig. 9 ). Downregulation of ARRB1 significantly inhibited cellular growth and proliferation in HepG2, Huh7 and LO2 lines ( Supplementary Fig. 4 ). These data confirmed that ARRB1 enhances inflammation-induced hepatocellular carcinogenesis by promoting hepatocellular malignant proliferation. TNF-α not only serves as a key mediator of hepatocyte apoptosis resulting in the liver damage, but also plays an important role in cellular proliferation leading to liver regeneration and even hepatocarcinogenesis in liver [39] . In this study, our results showed that TNF-α treatment significantly induced ARRB1 expression in both human HCC cell lines and mice hepatic tissues ( Fig. 7 ) and suggested that TNF-α may be an essential promotor of ARRB1 expression. Other studies have shown that ARRB1 is involved in several types of cancer by serving as a scaffold protein in various signal pathways, including ERK1/2, Wnt/β-catenin and c-Src [25] . Previous studies have established that ARRB1 is involved in cell proliferation, apoptosis and differentiation by mediating Akt phosphorylation response to a wide range of stimuli in different cell types [28] , [40] . Akt is essential for HCC development in both mice and humans, and HCC samples have revealed that activation of Akt is associated with poor prognosis [41] . We investigated the molecular mechanism of ARRB1 involved in hepatocellular carcinogenesis. The data showed that ARRB1 overexpression clearly promoted Akt phosphorylation (active form) and PCNA upregulation in vitro , whereas ARRB1 knockdown clearly depressed Akt phosphorylation and PCNA expression. Furthermore, the Akt inhibitor A6730 significantly repressed ARRB1-induced PCNA upregulation ( Fig. 8 ). In addition, our results showed that ARRB1- KO mice had clearly depressed hepatic Akt phosphorylation and downregulated PCNA expression 10 days after DEN treatment ( Fig. 10 ), and ARRB1- KO mice also had markedly depressed Akt activity and PCNA expression in both HCC tissues and its paracancerous tissues 9 months after DEN treatment ( Supplementary Fig. 5 ). In human HCC samples, upregulation of ARRB1 expression was linked with Akt phosphorylation ( Supplementary Fig. 6 ). Akt has been established as an important modulator of hepatocellular carcinoma. In this study, we demonstrated that ARRB1 interacts with Akt, thus providing a solid basis for ARRB1/Akt signalling. Our study further revealed that the ARRB1 interaction with Akt was significantly promoted by inflammatory stimulation with TNF-α ( Fig. 10e,f ). Accordingly, the current study strongly suggests a potential role for TNF-α in the modulation of Akt-mediated hepatocellular carcinogenesis and clearly indicates that ARRB1 may serve as a signalling linker between the TNF-α and Akt pathways. Consequently, inflammation induces hepatocellular carcinogenesis via TNF-α-mediated ARRB1 interaction with Akt to drive hepatocellular malignant proliferation. Tissue samples and cell lines Seven normal liver tissue samples were from parahemangioma sites of hepatic hemangioma patients without hepatitis, and the paired tissue samples from HCC and paracancerous tissues were obtained from 89 hepatitis B virus-infected HCC patients during operations before any therapeutic intervention. All of the samples were subsequently verified by histology. The study protocol was approved by the Clinical Research Ethics Committee of The Third Affiliated Hospital of Sun Yat-Sen University. Written informed consent was received from each patient and healthy volunteers before inclusion in the study. HepG2 and Hep3B cell lines were obtained from the American Type Culture Collection (ATCC, Manassas, VA, USA). The cell lines were used in the study after negative testing for contamination with mycoplasma. The cells were cultured in Dulbecco’s modified Eagle’s medium (DMEM) for HepG2, Hep3B and Huh7 cell lines or RPMI 1640 medium for LO2 cell line (Gibco BRL, Rockville, MD, USA) with 10% fetal bovine serum. Cell lines (HepG2 and LO2) were treated with 10 μmol l −1 of the Akt kinase inhibitor A6730 for 2 h (Sigma, St Louis, MO, USA). Mice The procedures for all animal experiments were approved by the Institutional Animal Care and Use Committee at The Third Affiliated Hospital of Sun Yat-Sen University. ARRB1 +/+ and ARRB1 −/− , ARRB2 +/+ and ARRB2 −/− littermates on C57BL/6 background were generated from heterozygote intercrosses (Kindly provided by Dr R. J. Lefkowitz, Duke University Medical Centre, Durham, NC, USA). Genotyping was performed as previously described [42] . The mice were housed in micro-isolator cages in a room illuminated from 0700 hours to 1900 hours (12:12-hour light/dark cycle) and were allowed access to water and chow ad libitum . Microarray experiment The Agilent SurePrint G3 Human Gene Expression 8 × 60 K Array was designed with eight identical arrays per slide, with each array containing probes interrogating about 27,958 Entrez Gene RNAs. The array also contains 1,280 Agilent control probes. The normal liver samples were obtained from normal hepatic tissue in three hepatic hemangioma surgical operative patients, and three matched pairs of HCC and its paracancerous tissues were, respectively, obtained from three HCC surgical operative patients without any chemotherapy and radiotherapy. The samples were subsequently verified by histology assay. Then, total RNA from each tissue sample was isolated according to the manufacturer’s instructions of TRIzol reagent (Invitrogen, Carlsbad, CA, USA) and was further purified with mirVana miRNA Isolation Kit (Ambion, Austin, TX, USA) according to the manufacturer’s protocol. The purity and concentration of RNA were determined from OD260/280 readings using spectrophotometer (NanoDrop ND-1,000). cDNA labelled with a fluorescent dye (Cy3-dCTP) was produced by Eberwine’s linear RNA amplification method and subsequent enzymatic reaction. This procedure has been improved using CapitalBio cRNA Amplification and Labelling Kit (CapitalBio, Beijing, China) for producing higher yields of labelled cDNA. After completion of double-stranded cDNA (dsDNA) synthesis using DNA polymerase and RNase H, the dsDNA products were purified using a PCR NucleoSpin Extract II Kit (MN) and eluted with 30 μl elution buffer. The eluted double-stranded cDNA products were vacuums evaporated to 16 μl and subjected to 40 μl in vitro transcription reactions at 37 °C for 14 h using a T7 Enzyme Mix. Klenow enzyme labelling strategy was adopted after reverse transcription using CbcScript II reverse transcriptase. Array hybridization was performed in a Agilent Hybridization oven overnight at a rotation speed of 20 r.p.m. at 42 °C and washed with two consecutive solutions (0.2% SDS, 2 × SSC at 42 °C for 5 min, and 0.2 × SSC for 5 min at room temperature). Details of the probe set can be obtained at http://www.chem.agilent.com/library/brochures/5989-3805EN.pdf . The array data were analysed for data summarization, normalization and quality control using the GeneSpring software V12 (Agilent). To select the differentially expressed genes, we used threshold values of ≥1.5 and ≤−1.5-fold change and a Benjamini-Hochberg-corrected P value of 0.05. The data were Log2 transformed and median centred by genes using the Adjust Data function of CLUSTER 3.0 software and then further analysed with hierarchical clustering with average linkage. Finally, tree visualization was performed using Java Treeview (Stanford University School of Medicine, Stanford, CA, USA). Accession number is available from the NCBI under GEO accession number (GSE67764). Treatment of mice Male mice were used in all study. For the diethylnitrosamine (DEN)-induced HCC model, DEN (15 mg kg −1 ) was intraperitoneally injected once into 15-day-old mice. Mice were killed after 9 months on standard diet. Surface tumour nodules in each liver lobe were counted and measured with a caliper. For study of tetrachloromethane (CCl 4 )-induced cirrhosis, 8-week-old mice were intraperitoneally injected with 20% CCl 4 (Sinopharm Chemical Reagent, China) dissolved in olive oil solution (Sinopharm Chemical Reagent, China) at 5 ml kg −1 body weight, twice per week for 8 weeks. The vehicle group was intraperitoneally injected with equivalent volume olive oil, twice per week for 8 weeks. For short-term studies of DEN-induced liver inflammation, 8- to 12-week-old mice were intraperitoneally injected with DEN dissolved in physiological saline at 100 mg kg −1 body weight and killed after 10 days. Mice receiving treatment with TNF-α (40 μg kg −1 ) were intraperitoneally injected twice 6 h before being killed. Mice receiving the Akt inhibitor (A6730, 50 mg kg −1 ) were intraperitoneally injected once 6 h before being killed. The vehicle treatment was intraperitoneal injection with equivalent volume physiological saline. MRI scan in DEN-induced HCC mice model The mice were anaesthetized for 1 h by intraperitoneal injection of 4% chloral hydrate (200 mg kg −1 ), and scanned by 3T MRI (TOSHIBA, Tokyo, Japan) using a T(2)-weighted sequence following intraperitoneal injection of contrast medium, gadobenate dimeglumine (Bracco Imaging, Milan, Italy) at a 0.1 mmol kg −1 dose. Total RNA extraction and real-time PCR Total RNA was isolated from the liver tissue samples using the RNAgents Total RNA Isolation System (Promega, Madison, WI, USA) according to the manufacturer’s instructions. First-strand cDNA was synthesized using Superscript Reverse Transcriptase (Invitrogen, Carlsbad, CA, USA) according to the manufacturer’s instructions. Real-time PCR was performed on a Chromo 4 Detector System (MJ Research, Sierra Point, CA, USA) using gene-specific primers and DyNAmo SYBR Green Master Mix (Finnzymes, Espoo, Finland). Real-time RT-PCR was performed using SYBR Green master mixture (Invitrogen, Carlsbad, CA, USA) on HT7500 system (Applied Biosystems). Primer sequences are listed in ( Supplementary Table 2 ). As the internal control, the expression of β-actin in each sample was also quantified. PCR products were analysed. Protein extraction and western blotting Total protein extractions were analysed by western blotting. Western blotting was performed using antibodies for ARRB1 (IB: 1:1,000, 1274-1) from Epitomics (Burlingame, CA, USA). Antibodies for PCNA (IB: 1:1,000, sc-56), ARRB2 (IB: 1:1,000, sc-13140), GFP (IB: 1:1,000, sc-8334) from Santa Cruz Biotechnology Inc (Santa Cruz, CA, USA). TNF-α (IB: 1:1,000, 3,707), Akt (IB: 1:1,000, 9,272), phospho-Akt (Ser473) (IB: 1:1,000, 4060) and cleaved caspase-3 (IB: 1:1,000, 9,661) obtained from Cell Signaling Technology (Danvers, MA, USA). Antibodies for PI3K (IB: 1:1,000, SAB4502195) and β-actin (IB: 1:7,000, A5441) were purchased from Sigma-Aldrich (St Louis, MO, USA). The signal was detected using ECL western blotting detection reagents (Amersham Pharmacia Biotech, Piscataway, NJ, USA). After quantifying the signals by densitometry, the results are expressed as a ratio to loading control densitometry units. Unedited images of IBs are shown in Supplementary Figs 7–11 . Immunoprecipitation The cells were lysed in lysis buffer (50 mM Tris-HCl, pH 7.5, 1 mM EDTA, 150 mM NaCl, 20 mM NaF, 0.5% Nonidet P-40, 10% glycerol, 1 mM phenylmethylsulfonyl fluoride) for 1.5 h at 4 °C at 48 h after transfection. The cell extracts were cleared, and the supernatant was incubated at 4 °C with anti-GFP (1 μg, Roche Molecular Biochemicals 11814460001) or anti-ARRB1 (1 μg, Santa Cruz Biotechnology sc-9182) antibody overnight. Immune complexes were immobilized on protein A (Amersham Biosciences) or anti-chicken IgY Sepharose beads (Promega) for 3 h, washed three times with lysis buffer and heated in SDS sample buffer in a 50 °C water bath for 20 min. Western blot analysis was performed as described above. GFP-tagged proteins were detected with an anti-GFP antibody. Endogenous Akt was detected with an antibody specific to Akt (Cell Signaling Technology). Immunohistological staining Sections were deparaffinized, rehydrated and treated with 3% hydrogen peroxide. Antigen retrieval was performed by boiling the sections for 2 min in Tris/EDTA Antigen Retrieval Solution (pH 9.0). Nonspecific antibody binding was blocked using 15% goat serum for 30 min. For staining in tissue samples, the slides were incubated with primary antibodies against ARRB1 (1:100, Epitomics 1274-1), MPO (1:200, Santa Cruz sc-59600), CD68 (1:200, Santa Cruz sc-20060), IL-6 (1:200, Santa Cruz sc-130326), PCNA (1:400, Santa Cruz sc-56), TNF-α (1:200, Santa Cruz sc-52746), cleaved caspase-3 (1:100, Cell Signaling 9,661), HA (1:400, Cell Signaling 2,367), phospho-Akt (1:200, Cell Signaling 4,060) and Ki-67 antibody (1:400, Abcam ab66155). For IHC staining, the targeted protein was detected using secondary antibodies followed by detection using the ABC staining system (Santa Cruz), and the sections were counterstained with haematoxylin. For IF staining, targeted proteins were detected by related secondary antibody. Antibody–antigen complexes were visualized by incubation with biotin-conjugated secondary antibody and streptavidin Alexa 488 (Molecular Probes, Eugene, OR, USA), with the nuclei counterstained with 2 mg ml −1 of 4’, 6-diamidino-2-phenylindole dihydrochloride (DAPI) (Molecular Probes). Terminal deoxynucleotidyl transferase-mediated dUTP-digoxigenin nick end labelling (TUNEL) assay was performed using an in situ cell death detection kit (Roche, Basel, Switzerland) according to the manufacturer’s instructions. Nuclei with clear brown staining were regarded as TUNEL-positive apoptotic cells. Cells with positive staining were measured by counting 1,000 cells in each sample and are reported as the mean±s.d. Cell growth and colony formation assay Cell growth was measured by the CCK-8 assay (Dojindo, Kumamoto, Japan). In brief, the cells (1 × 10 3 /well) were stably transfected with pcDNA3.0- ARRB1-GFP , pcDNA3.0- GFP vector or transfected with ARRB1-siRNA, control-siRNA in a 96-well plate for 24 to 96 h. WST-8 reaction solution (20 μl) was added to cells in 180 μl culture medium, incubated at 37 °C for 3 h and measured at a wavelength of 450 nm. Colony formation assay was performed using monolayer culture. Cells (4 × 10 5 /well) were plated in a six-well plate and transfected with expression plasmids pcDNA3.0- ARRB1 -GFP, pcDNA3.0- ARRB1 -HA, pcDNA3.0- ARRB2 -HA, pcDNA3.0-GFP or pcDNA3.0-HA vector (2 μg in each) (Kindly provided by Dr Pei G, Chinese Academy of Sciences, Shanghai) using lipofectamine 2000 (Invitrogen). After 48 h of transfection, the cells were collected and seeded (1 × 10 4 /well) in a fresh six-well plate and selected with G418 for 10 days. Colonies containing more than 50 cells were counted after staining with crystal violet solution. All of the experiments were performed in triplicate wells and repeated three times. Small interfering RNA Small interfering RNA (siRNA) was performed according to the manufacturer’s instructions. Cells were cultured in six-well plates. For ARRB1 siRNA treatment, cells were transfected with 20 μM ARRB1 RNA oligo kit (Gene Pharma, China). The ARRB1 siRNA sequence targeted the coding region of the ARRB1 mRNA ( Supplementary Table 3 ). All of the experiments were performed in triplicate wells and repeated three times. MPO activity assay Mice liver specimens were homogenized in 0.5% hexadecyltrimethylammonium bromide dissolved in 50 mM phosphate buffer (pH 6.0) and sonicated for 10 s. Suspensions were freeze-thawed three times, and then centrifuged at 15,000 r.p.m. for 15 min. Supernatant of 100 μl was mixed with a solution of 0.167 mg ml −1 O-dianisidine hydrochloride and 0.0005% hydrogen peroxide. MPO activity was measured spectrophotometrically as the change in absorbance at 460 nm. Xenograft tumours Xenograft tumours were established by subcutaneous injection of 5 × 10 6 Hep3B cells into both flanks of 6-week-old male Balb/c athymic nude mice ( n =5, in each). Hep3B cells were stably overexpressed with pcDNA3.0- ARRB1-HA or pcDNA3.0- ARRB2-HA and pcDNA3.0 -HA vector. The athymic nude mice were purchased from animal centre of Sun Yat-Sen University (Guangzhou, China). Tumour growth was monitored by calipers every 3 days after inoculation. The tumour volume was calculated according to the formula (0.5 × length × width 2 ). Statistical analysis Statistical analysis was performed using GraphPad Prism V software. Data are presented as means±s.d.. Statistical significance was calculated with the independent Student’s t test for protein expression, comparing cellular proliferation, colony formation, gene expression and tumorigenicity between two selected groups. χ 2 -test is used to analyse the positive rate differences among human normal liver tissues and human HCC specimens as well as its paracancerous samples. The transcript levels of ARRB1 in human normal liver, paracancerous and HCC tissues were compared using one-way ANOVA test. Differences were considered to be significant if the probability of the difference occurring by chance was <5 in 100 ( P <0.05). How to cite this article: Yang, Y. et al. β-arrestin1 enhances hepatocellular carcinogenesis through inflammation-mediated Akt signalling. Nat. Commun. 6:7369 doi: 10.1038/ncomms8369 (2015).